De novo design of Au36(SR)24nanoclusters The discovery of atomically precise nanoclusters is generally unpredictable, and the rational synthesis of nanoclusters guided by the theoretical design is still in its infancy. Here we present a de novo design of Au 36 (SR) 24 nanoclusters, from theoretical prediction to experimental synthesis and characterization of their physicochemical properties. The crystal structure of an Au 36 (SR) 24 nanocluster perfectly matches the simulated structural pattern with Au 4 tetrahedral units along a two-dimensional growth. The Au 36 (SR) 24 nanocluster indeed differs from its structural isomer whose kernel is dissected in an Au 4 tetrahedral manner along a one-dimensional growth. The structural isomerism in the Au 36 (SR) 24 nanoclusters further induces distinct differences in ultrafast electron dynamics and chirality. This work will not only promote the atomically precise synthesis of nanoclusters enlightened by theoretical science, but also open up exciting opportunities for underpinning the widespread applications of structural isomers with atomic precision. Thiolate-protected atomically precise gold nanoclusters referred to as Au n (SR) m ( n = gold atom number; m = ligand number) constitute a generation of gold nanoparticles and exhibit unique physical and chemical properties in optics, electronics, catalysis, chirality, and sensing [1] , [2] , [3] , [4] , [5] , [6] , [7] , [8] , [9] . Since the total structure of Au 102 (SR) 44 was resolved [10] , the synthesis of one pot for one size starts to bloom and gold nanoclusters are constantly springing up [11] , [12] , [13] , [14] , [15] , [16] , [17] , [18] . However, despite the significant advances in Au n (SR) m nanocluster studies, several critical issues remain still unclear, e.g. what exactly determines the structure of nanoclusters and what are real growth behaviors of nanoclusters in the solution phase? Moreover, whether the experimentalists can synthesize the specific nanoclusters based on the theoretical design is still challenging. In this work, we first identify the most potential candidate of Au n (SR) m nanoclusters by the grand unified model (GUM) and density functional theory (DFT) calculations. Further we synthesize this nanocluster and prove its distinct property in optics and chirality. The work demonstrates the feasibility of rational synthesis of nanoclusters based on de novo design. In correlating the conventional characterization information with the growth mechanism of nanoclusters, extensive studies have been applied to the combination of experimental and theoretical results to explore the growth of the basic structural units into smart structures [19] , [20] , [21] , [22] , [23] , [24] , [25] , [26] , [27] , [28] . Among these works, Au 4 tetrahedron identified as a building block can be assembled into a series of Au n (SR) m nanoclusters [20] , [21] , [29] , [30] , [31] , [32] , [33] . Especially, the solved crystal structures of a periodic series with a unified formula of Au 8 n +4 (TBBT) 4 n +8 (TBBT = 4-tert-butylbenzenethiol, n = 3–6) nanoclusters reflect that their kernels are adopted in the connection mode of Au 4 tetrahedron along one dimension [32] . It should be noted that Au 28 (CHT) 20 (the isomer of Au 28 (TBBT) 20 to some extent, cyclohexanethiol (CHT)) also contains the one-dimensional Au 14 kernel made up of Au 4 units. Recently, the discovery of structural isomerism in the Au 52 (SR) 32 provided the first example that the kernel of Au 52 (SR) 32 isomer can be arranged in a two-dimensional growth of Au 4 tetrahedra [33] . A question naturally is whether the Au 4 tetrahedron-based two-dimensional growth mode can be further extended to hitherto non-synthesized isomers in the family of Au 8 n +4 (SR) 4 n +8 . To address this, we initiate theoretical studies to predict the structures of a series of Au 8 n +4 (SR) 4 n +8 with Au 4 tetrahedron as the building unit in a two-dimensional growth pattern. Subsequently, we identify an Au 36 (SR) 24 packed in two-dimensional mode that has the highest stability among all the isomers, which would be an ideal candidate for experimental synthesis to fill in one of missing isomers in the family. By calculation-assisted nanoclusters discovery, a couple of isomeric Au 36 (SR) 24 nanoclusters protected by 3,5-dimethylbenzenethiol (DMBT) are successfully synthesized and their crystal structures accurately match the predicted ones. The Au 36 (DMBT) 24 nanocluster packed in two-dimensional mode is chiral, whereas the other isomer whose structure is identical to the previously reported Au 36 (TBBT) 24 is achiral. The two Au 36 (DMBT) 24 nanoclusters also exhibit dramatic differences in ultrafast dynamics. Theoretical prediction Based on GUM, there is a potential two-dimensional growth pattern, in which the growth of gold kernels in thiolate-protected gold nanoclusters can be viewed as the sequent addition of elementary blocks (tetrahedral Au 4 in this case) obeying duet rule [21] , [28] . As shown in Fig. 1 , there are two types of face-centered cubic (fcc) growth pattern for the kernels of Au 8 n +4 (SR) 4 n +8 ( n = 3, 4, 5, 6) using Au 4 building blocks. Starting from the predicted Au 28 (SR) 20 (a3 in Fig. 1 ) [22] , two Au 4 units are fused with the Au 14 kernel of Au 28 (SR) 20 (a3 in Fig. 1 ) by sharing two gold atoms to form a new Au 20 kernel, resulting in two Au 36 (SR) 24 isomers (b2 and b3 in Fig. 1 ). Continuing fusing two Au 4 units with the Au 20 kernel of Au 36 (SR) 24 can form an Au 44 (SR) 28 isomer with Au 26 kernel (c2 in Fig. 1 ). Following the same way, two different Au 32 kernels can be obtained to form two Au 52 (SR) 32 isomers (d2 and d3 in Fig. 1 ). Among them, the d2 of Au 52 (SR) 32 protected by 2-phenylethanethiol (denoted as PET) was experimentally determined [33] . In this work, as illustrated in Fig. 1 , totally four new isomers for Au 8 n +4 (SR) 4 n +8 series have been theoretically predicted based on GUM. The series follow the two-dimensional growth mode (green arrows in Fig. 1 ), which is completely different from the one-dimensional double-helical growth for old series (blue arrows in Fig. 1 ). Fig. 1: The growth patterns of Au 8 n+4 (SR) 4n+8 ( n = 3–6) nanoclusters. The values in brackets are the relative energies (eV). Note that structures of a1/b1/c1/d1 (TBBT as ligand) and a2 (CHT as ligand) are experimentally determined. The arrows in blue and green denote the one-dimensional and two-dimensional growth, respectively. According to the relative energies, b2 of Au 36 (SR) 24 and d2 of Au 52 (SR) 32 are the most potential candidates among the predicted isomers. Color labels: green = S, blue/magenta/yellow = Au. The C and H atoms are omitted for clarity. Full size image All the predicted isomers (–R group is replaced by –H) were fully optimized using DFT method implemented in the Gaussian 09 program package [34] , including the TPSS functional [35] and the all-electron basis set 6–31 G* for H and S, effective-core basis set LANL2DZ for Au. Among the predicted isomers shown in Fig. 1 , the isomer b2 of Au 36 (SR) 24 is only 0.11 eV higher in energy than b1, implying that this structure may be stable and accessible. 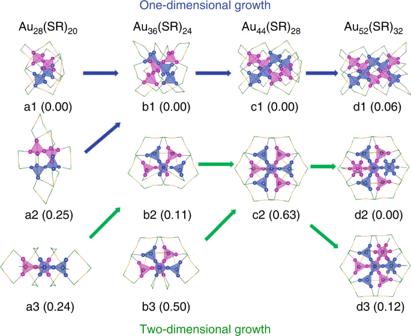Fig. 1: The growth patterns of Au8n+4(SR)4n+8(n= 3–6) nanoclusters. The values in brackets are the relative energies (eV). Note that structures of a1/b1/c1/d1 (TBBT as ligand) and a2 (CHT as ligand) are experimentally determined. The arrows in blue and green denote the one-dimensional and two-dimensional growth, respectively. According to the relative energies, b2 of Au36(SR)24and d2 of Au52(SR)32are the most potential candidates among the predicted isomers. Color labels: green = S, blue/magenta/yellow = Au. The C and H atoms are omitted for clarity. In addition, this cluster has a large HOMO–LUMO (HOMO/LUMO: the highest/lowest occupied/unoccupied molecular orbital) gap and all positive harmonic vibrational frequencies (Supplementary Table 1 ), indicating its thermal and chemical stability. Thus, it motivates us to synthesize this most potential candidate based on the GUM-guided prediction. Synthesis and characterization The b1 and b2 isomers in Au 36 (SR) 24 can be simultaneously synthesized using a two-step size-focusing method when DMBT was selected as the protected ligand. The two nanoclusters were denoted as Au 36 (DMBT) 24 -1D and Au 36 (DMBT) 24 -2D according to the growth modes (vide infra). Electrospray ionization mass spectra (ESI-MS) showed the m / z 5192.02 peak with +2 charge for both nanoclusters (Supplementary Fig. 1 ), corresponding to [Au 36 (DMBT) 24 -2e] 2+ (calculation: 5192.09 Da; deviation: 0.07 Da). The observed isotopic distributions were in perfect agreement with the simulated ones, further verifying the accurate formula of Au 36 (DMBT) 24 nanoclusters. 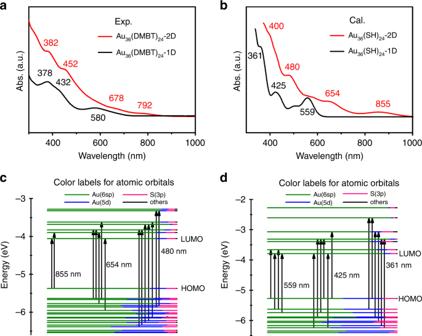Fig. 2: The optical absorption properties of Au36(DMBT)24nanoclusters. aExperimental UV-vis spectra of Au36(DMBT)24-2D and Au36(DMBT)24-1D.bCalculated UV-vis spectra of Au36(SH)24-2D and Au36(SH)24-1D. The values in the black or red are the wavelength (nm) corresponding to the absorption peaks. Molecular orbital (MO) energy level diagrams forcAu36(SH)24-2D anddAu36(SH)24-1D. The energies are in eV. Various colors are used to mark relative contributions (line length with color labels) of different orbitals. The major orbital contributions from the Au(6sp), Au(5d), and S(3p) are in olive, blue, and pink, respectively. The values in the black are the wavelength (nm) corresponding to the absorption peaks. Figure 2a showed the optical absorption spectra of Au 36 (DMBT) 24 . Au 36 (DMBT) 24 -2D exhibited the two-step peaks at 382 and 452 nm and two broad peaks at 678 and 792 nm, respectively, while Au 36 (DMBT) 24 -1D showed the two distinct peaks at 378 and 580 nm and one shoulder peak at 432 nm. The calculated UV-vis spectra of Au 36 (SH) 24 -2D and Au 36 (SH) 24 -1D were presented in Fig. 2b to reproduce the experimental results using linear response time-dependent density functional theory (TDDFT). The lowest 450 singlet-to-singlet excitation states were evaluated. As shown in Fig. 2b , the theoretical spectra can well reproduce the results of experimental measurements. Four absorption peaks (400, 480, 654, and 855 nm) for Au 36 (SH) 24 -2D and three absorption peaks (361, 425, and 559 nm) for Au 36 (SH) 24 -1D can be observed. Further examination of the Kohn–Sham (KS) molecular orbital (MO) energy levels and atomic orbital components in each KS MO of Au 36 (SH) 24 -2D and Au 36 (SH) 24 -1D indicate that the absorption peaks mainly involve the Au( sp ) → Au( sp ) transitions (Fig. 2c, d ). Accordingly, the optical energy gaps were determined to be 1.36 eV for Au 36 (DMBT) 24 -2D and 1.71 eV for Au 36 (DMBT) 24 -1D based on the photon-energy scaled spectra (Supplementary Fig. 2 ), which were consistent with the corresponding calculated values of 1.31 and 1.74 eV (Supplementary Table 1 ). Fig. 2: The optical absorption properties of Au 36 (DMBT) 24 nanoclusters. a Experimental UV-vis spectra of Au 36 (DMBT) 24 -2D and Au 36 (DMBT) 24 -1D. b Calculated UV-vis spectra of Au 36 (SH) 24 -2D and Au 36 (SH) 24 -1D. The values in the black or red are the wavelength (nm) corresponding to the absorption peaks. Molecular orbital (MO) energy level diagrams for c Au 36 (SH) 24 -2D and d Au 36 (SH) 24 -1D. The energies are in eV. Various colors are used to mark relative contributions (line length with color labels) of different orbitals. The major orbital contributions from the Au(6sp), Au(5d), and S(3p) are in olive, blue, and pink, respectively. The values in the black are the wavelength (nm) corresponding to the absorption peaks. Full size image Single-crystal X-ray crystallography studies showed that Au 36 (DMBT) 24 -2D can be divided into a 20-atom gold kernel and eight external staple motifs (Figs. 3 a and 4a ). Twenty gold atoms in the kernel can be further viewed as two groups of Au 4 tetrahedron which are arranged in a staggered mode, and this packing mode is in excellent agreement with the predicted two-dimensional growth (b2 in Fig. 1 ). The surface staple motifs can be divided into three categories: two monomeric Au 1 (SR) 2 , two trimeric Au 3 (SR) 4 , and four dimeric Au 2 (SR) 3 (Figs. 3 a and 4a ). Note that both Au 3 (SR) 4 and Au 2 (SR) 3 staples are not in a plane (Supplementary Fig. 3 ). Alternatively, after cutting the gold atoms from Au 1 (SR) 2 and Au 3 (SR) 4 staples, the remaining 28 gold atoms can be constructed in a layer-by-layer fashion, which respectively consists of 6/8/8/6 atoms (Supplementary Fig. 4 ). This fashion is akin to a fcc structure of previously reported gold nanoclusters [11] , [32] , [33] . Fig. 3: Crystal structures of the Au 36 (DMBT) 24 nanoclusters. Structural frameworks of a Au 36 (DMBT) 24 -2D and b Au 36 (DMBT) 24 -1D shown in tetrahedral Au 4 networks. Color labels: yellow = S, blue/magenta/green = Au. The C and H atoms are omitted for clarity. Full size image Fig. 4: Comparison of the Au 36 (DMBT) 24 structures. Structural frameworks of a Au 36 (DMBT) 24 -2D and b Au 36 (DMBT) 24 -1D shown in stacking mode. Color labels: yellow = S, blue/magenta/red = Au. The C and H atoms are omitted for clarity. Full size image As the counterpart of Au 36 (DMBT) 24 -2D, Au 36 (DMBT) 24 -1D adopts a totally different configuration from Au 36 (DMBT) 24 -2D, although it owns a 20-Au-atom kernel as well. In fact, the helical tetrahedron in the Au 36 (DMBT) 24 -1D is along the one-dimensional growth (Figs. 3 b and 4b ), in contrast to Au 36 (DMBT) 24 -2D (Figs. 3 a and 4a ), which are excellently consistent with the growing modes of the predicted b1 and b2 of Au 36 (SR) 24 nanoclusters (Fig. 1 ). Notably, the Au 36 (SR) 24 -1D and Au 36 (SR) 24 -2D can be described by superatom network (SAN) model [26] with using the adaptive natural density partitioning (AdNDP) analysis [36] on the Au 20 8+ of both Au 36 (SR) 24 , which show the 12e valence electrons of Au 36 (SR) 24 are equally distributed on six tetrahedral Au 4 units, respectively (Supplementary Fig. 5 ). Thus, the Au 20 core of each Au 36 (SR) 24 can be viewed as a network of six 4c-2e (4c denotes 4 centers). Another notable issue is that the structural framework of Au 36 (DMBT) 24 -1D is identical to that of reported Au 36 (TBBT) 24 [11] . There are four non-planar and four co-planar staple motifs Au 2 (SR) 3 in Au 36 (DMBT) 24 -1D (Supplementary Fig. 3 ). After cutting the Au atoms from co-planar Au 2 (SR) 3 staples, the remaining 28 Au atoms of Au 36 (DMBT) 24 -1D are packed in a fcc structure (Supplementary Figs. 6 and 7 ). As we know, the previous studies showed the non-fcc vs. non-fcc isomerization appeared in the Au 38 (PET) 24 isomers and the fcc vs. non-fcc isomerization existed in the Au 42 (TBBT) 26 isomers [15] , [37] . Here the fcc vs. fcc isomerization is for the first time observed in the Au 36 (DMBT) 24 isomers. In addition, Au 36 (DMBT) 24 -2D can be irreversibly converted to Au 36 (DMBT) 24 -1D at 333 K for 2 h, which indicates that the latter is more stable than the former. To further corroborate the mechanism of two-dimensional growth in the series of Au 8 n +4 (SR) 4 n +8 nanoclusters, we tried to synthesize c2 isomer of Au 44 (SR) 28 using various synthetic methods, e.g., one-pot reduction, size-focusing, and thermal conversion (the synthesis details are shown in Methods section). Different ligands were employed such as 3-methylbenzenethiol, 4-isopropylbenzenethiol, 2,4-dimethylbenzenethiol, etc. 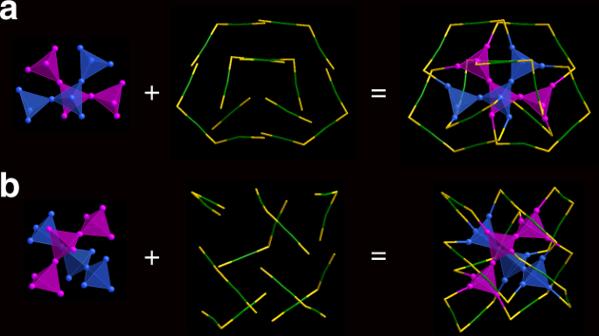Fig. 3: Crystal structures of the Au36(DMBT)24nanoclusters. Structural frameworks ofaAu36(DMBT)24-2D andbAu36(DMBT)24-1D shown in tetrahedral Au4networks. Color labels: yellow = S, blue/magenta/green = Au. The C and H atoms are omitted for clarity. The experimental conditions were controlled by tuning temperature and pH in different solvents. Under the above attempts, we obtained Au 36 (SR) 24 -1D, Au 44 (SR) 28 -1D, and other unknown nanoclusters, which were indicated by UV-vis (Supplementary Fig. 8 ) and ESI-MS spectra (Supplementary Figs. 9 and 10 ). The c2 isomer of Au 44 (SR) 28 (denoted as Au 44 (SR) 28 -2D) was not obtained, which is possibly because the Au 44 (SR) 28 -2D (0.63 eV) is notably higher in energy than Au 44 (SR) 28 -1D (0 eV) (Fig. 1 ). In addition, as is known, the synthesis of nanoclusters involves kinetic control in the early stage and the carbon tail of the thiol ligands often plays an important role. While we believe the Au 44 (SR) 28 -2D would be attainable, their syntheses might take an exhaustive search for the right HS-R to reach the exact conditions. Therefore, we have to leave this to future work. 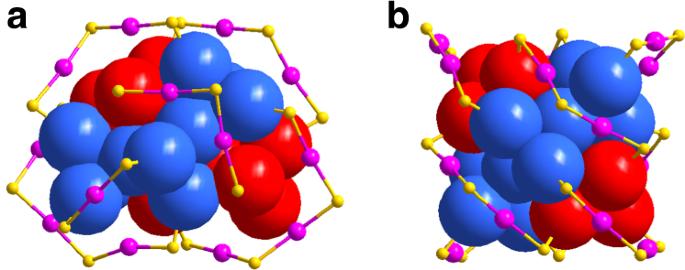Fig. 4: Comparison of the Au36(DMBT)24structures. Structural frameworks ofaAu36(DMBT)24-2D andbAu36(DMBT)24-1D shown in stacking mode. Color labels: yellow = S, blue/magenta/red = Au. The C and H atoms are omitted for clarity. Notably, the d2 isomer of Au 52 (SR) 32 can be synthesized with the assistance of acid [33] . The Au 32 kernel of Au 52 (TBBT) 32 (d1 isomer) adopts the one-dimensional growth of the Au 4 units (Supplementary Fig. 11a ) [32] , while the kernel of Au 52 (PET) 32 (d2 isomer) consists of 32 gold atoms that are arranged along two-dimensional direction based on the Au 4 tetrahedron (Supplementary Fig. 11b ). Thus, the Au 52 (PET) 32 nanocluster further supports the possibility of the two-dimensional growth for Au 4 units of Au 8 n +4 (SR) 4 n +8 proposed in this work. Chirality Au 36 (DMBT) 24 -2D is chiral, as the Au 20 kernel and surface staple units are both arranged in a chiral pattern (Fig. 5a ), while Au 36 (DMBT) 24 -1D is achiral due to no mirror plane occurring in the metal kernel and the surface staples (Figs. 3 b and 4b ). We separated the Au 36 (DMBT) 24 -2D enantiomers by high-performance liquid chromatography (HPLC) (Supplementary Fig. 12 ) and studied its chirality by circular dichroism (CD) [38] , [39] , [40] , [41] , [42] . 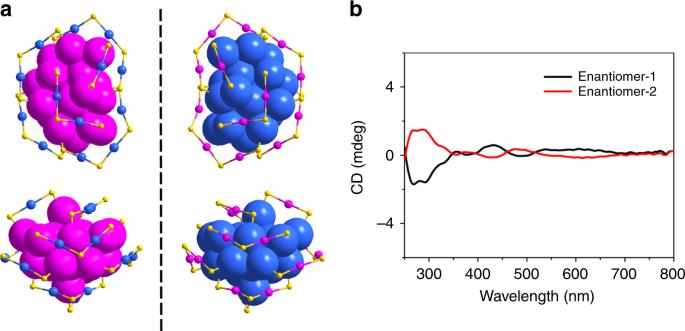Fig. 5: Chirality of the Au36(DMBT)24-2D nanocluster. aThe enantiomers of Au36(DMBT)24-2D from top view (upper panel) and side view (lower panel). Color labels: yellow = S, blue/magenta = Au. The C and H atoms are omitted for clarity.bCD spectra of the separated enantiomers of Au36(DMBT)24-2D. As shown in Fig. 5b , the pair of Au 36 (DMBT) 24 -2D enantiomers showed a mirror symmetry for multiple peaks in the CD spectra, which were respectively centered at 268, 292, 329, 355, 380, 430, 487, and 615 nm in the UV-vis spectral region. The theoretically simulated CD spectra for Au 36 (SH) 24 enantiomers agreed with the experimental spectra (Supplementary Fig. 13 ). Fig. 5: Chirality of the Au 36 (DMBT) 24 -2D nanocluster. a The enantiomers of Au 36 (DMBT) 24 -2D from top view (upper panel) and side view (lower panel). Color labels: yellow = S, blue/magenta = Au. The C and H atoms are omitted for clarity. b CD spectra of the separated enantiomers of Au 36 (DMBT) 24 -2D. Full size image Ultrafast electron dynamics The dynamics of excited states in the two Au 36 (DMBT) 24 nanoclusters were studied by using transient absorption (TA) spectroscopic measurements. 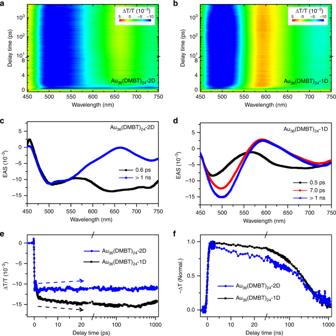Fig. 6: Excited-state dynamics of Au36(DMBT)24nanoclusters. Femtosecond-resolved transient absorption data recorded fromaAu36(DMBT)24-2D andbAu36(DMBT)24-1D. Spectral features of different delay components derived from global fitting analysis forcAu36(DMBT)24-2D anddAu36(DMBT)24-1D.eFemtosecond-resolved andfnanosecond-resolved dynamic traces of the two nanoclusters. Figure 6a, b compared the femtosecond-resolved TA data of two isomers pumped at 400 nm. We carried out the global fitting analysis to extract the evolution associated spectra (EAS) of the isomers, as shown in Fig. 6c, d . Except for some slight wavelength shifted, the spectral characteristics showed similar features for both nanoclusters with excited-state absorption near 500 nm and ground-state bleach near 600 nm, respectively. Nonetheless, the temporal dynamics exhibited remarkable differences for the two isomers. For the Au 36 (DMBT) 24 -1D nanocluster, the experimental data can be reproduced by three processes with lifetime parameters of 0.5 ps, 7 ps, and >1 ns (Fig. 6d ), respectively. In analogy to the previously reported results on Au 36 (TBBT) 24 nanocluster, the three components can be attributed to ultrafast S n → S 1 internal conversion, structural relaxation, and carrier recombination, respectively [43] . However, the component of structural relaxation (~ 7 ps) was not present in the data recorded from the Au 36 (DMBT) 24 -2D nanocluster (Fig. 6c ). Such a difference was explicitly manifested in the dynamics probed at 500 nm (Fig. 6e ; more meticulous comparison shown in Supplementary Fig. 14 ), where a delayed rise in the excited-state absorption signal observed from the Au 36 (DMBT) 24 -1D sample was absent in the data recorded from the Au 36 (DMBT) 24 -2D sample. This marked difference between the electron dynamics in the two isomers is probably related to their different structures: the picosecond component with lifetime of ~7 ps in Au 36 (DMBT) 24 -1D nanoclusters is the structural relaxation due to the expansion or torsion of one-dimensional chains after excitation [43] , while the ~7 ps component is not observed in Au 36 (DMBT) 24 -2D nanoclusters, which may be due to the limitation of the conformation changes in the two-dimensional kernel. In addition, it was found that the carrier recombination in the Au 36 (DMBT) 24 -2D sample became slightly faster than that in the Au 36 (DMBT) 24 -1D sample (Fig. 6f ). These observations are interesting that Au 36 (DMBT) 24 -2D and Au 36 (DMBT) 24 -1D have same chemical compositions, but show drastic differences in their optical features and electron dynamics. Fig. 6: Excited-state dynamics of Au 36 (DMBT) 24 nanoclusters. Femtosecond-resolved transient absorption data recorded from a Au 36 (DMBT) 24 -2D and b Au 36 (DMBT) 24 -1D. Spectral features of different delay components derived from global fitting analysis for c Au 36 (DMBT) 24 -2D and d Au 36 (DMBT) 24 -1D. e Femtosecond-resolved and f nanosecond-resolved dynamic traces of the two nanoclusters. Full size image On the basis of the theoretical prediction for decision making, we have successfully synthesized a pair of isomeric Au 36 (DMBT) 24 nanoclusters by selecting an appropriate ligand: one is constructed from Au 4 tetrahedral units along the two-dimensional growth, whereas the other is patterned in an Au 4 tetrahedral manner along the one-dimensional growth. The isomerism in the two Au 36 (DMBT) 24 nanoclusters indeed induces evident differences in physicochemical properties, such as optics, chirality, and ultrafast dynamics. This de novo design of Au 36 (SR) 24 is expected to stimulate further work on the synthetic chemistry guided by theoretical studies as well as on the practical applications of atomically precise isomeric nanoclusters. Materials All chemicals and reagents are commercially available and used without further purification. 3,5-dimethylbenzenethiol (3,5-DMBT, 98.0%), 4-tert-butylbenzenethiol (TBBT, 98.0%), 4-methylbenzenethiol (4-MBT, 98.0%), 3-methylbenzenethiol (3-MBT, 97.0%), 4-ethylbenzenethiol (4-EBT, 97.0%), 4-isopropylbenzenethiol (4-IPBT, 96.0%), 2,4-dimethylbenzenethiol (2,4-DMBT, 95.0%), 2-phenylethanethiol (PET, 97.0%), 4-tert-butyl benzyl mercaptan (97.0%), benzyl mercaptan (98.0%), and tetra-octylammonium bromide (TOAB, 98.0%) were purchased from Aladdin. Tetrachloroauric (III) acid (HAuCl 4 ∙ 4H 2 O, 99.9%), sodium borohydride (NaBH 4 , 98.0%), methanol (CH 3 OH, 99.5%), dichloromethane (CH 2 Cl 2 , 99.0%), acetonitrile (CH 3 CN, 99.0%), toluene (PhCH 3 , 99.5%), and petroleum ether (AR) were obtained from Sinopharm Chemical Reagent. Co. Ltd. The water used in all experiments was ultrapure with the resistivity of 18.2 MΩ∙cm produced by a Milli-Q NANO pure water system. Synthesis of Au 36 (DMBT) 24 nanoclusters Au 36 (DMBT) 24 -2D and Au 36 (DMBT) 24 -1D nanoclusters were simultaneously synthesized using a two-step size-focusing method. Step 1: 50 mg of HAuCl 4 ∙ 4H 2 O (0.12 mmol) dissolved in 1 mL water was mixed with 10 mL CH 2 Cl 2 containing TOAB (80 mg, 0.15 mmol). After vigorously stirring for 20 min, the organic layer was transferred into a 50-mL flask and 60-μL 3,5-dimethylbenzenethiol (DMBT) was injected. The above mixture was stirred until the color of the solution was clear, then an aqueous solution containing 25 mg of NaBH 4 was added at once. The reduction was allowed to proceed for 6 h. After that, the reaction mixture was dried by a rotary evaporator, and the obtained precipitates were washed with methanol three times to remove excess ligands and salts. Step 2: the obtained precursor was extracted with 0.5 mL toluene and then etched by 0.5 mL DMBT for 48 h at room temperature. The crude product was washed with CH 3 OH and separated by thin-layer chromatography. Both Au 36 (DMBT) 24 -2D and Au 36 (DMBT) 24 -1D nanoclusters were crystallized in toluene/acetonitrile solution by vapor diffusion over two weeks. Synthetic attempts for Au 44 (SR) 28 -2D nanoclusters (1) Size-focusing method: the nanoclusters were prepared from the ligand (4-methylbenzenethiol, 3-methylbenzenethiol, 4-ethylbenzenethiol, 4-isopropylbenzenethiol, or 4-tert-butylphenylthiol) in place of DMBT under otherwise identical experimental conditions of Au 36 (DMBT) 24 mentioned above. (2) One-pot reduction method: 50 mg of HAuCl 4 ∙4H 2 O (0.12 mmol) and 100 mg of TOAB were dissolved in 17 mL solvent such as tetrahydrofuran, dichloromethane, or ethyl acetate. After vigorously stirring for 20 min, 190 μL organic ligand (e.g., benzyl mercaptan, 3,5-dimethylbenzenethiol, 2,4-dimethylbenzenethiol, 4-tert-butyl benzyl mercaptan, or 2-phenylethanethiol) was injected. The above mixture was stirred until the color of the solution was clear (~2 h), and then the pH was adjusted by adding H + or OH − prior to reduction. An aqueous solution containing 60 mg of NaBH 4 was added in the above mixture at once and the reduction was allowed to proceed for ~14 h. After that, the solution was evaporated and the residue was washed with CH 3 OH for three times. Finally, the product was separated by thin-layer chromatography. (3) Thermal conversion method: e.g., 20 mg of Au 44 (DMBT) 28 -1D was dissolved in 2 mL toluene and 2 mL 2,4-dimethylbenzenethiol. The mixture was maintained at 60 °C for 24 h. The crude product was washed with CH 3 OH and separated by thin-layer chromatography. X-ray crystallography The single-crystal X-ray diffraction data for Au 36 (DMBT) 24 -2D and Au 36 (DMBT) 24 -1D nanoclusters were collected on a Bruker D8 VENTURE using Mo Kα radiation ( λ = 0.71073 Å) and Ga Kα radiation ( λ = 1.34139 Å), respectively. The structure was solved by ShelxT and refined by ShelxL. Platon-Squeeze program was used to remove the contributions of disordered solvent. Chirality measurements The enantiomers of Au 36 (DMBT) 24 -2D were separated by HPLC on a DIONEX UltiMate 3000 system (Thermo SCIENTIFIC) equipped with Chiral AS column (DAICEL), where the mobile phase was isopropanol/hexane = 2/98, the flow rate was set at 0.5 mL min −1 and the eluents were collected at different times. CD spectra were carried out on CD JASCO J-810 and the enantiomers were dissolved in dichloromethane for CD measurements. Ultrafast optical measurements A Ti:sapphire regenerative amplifier (Libra, Coherent Inc.) was used for TA spectroscopy. For femtosecond TA experiment, the optical delay between the pump and probe beams was enabled by a translation stage. The pump beam at 400 nm wavelength was from the second harmonic generation of BBO crystal pumped by a portion of laser from the regenerative amplifier. The probe beam was a broadband supercontinuum light source generated by focusing a small portion of the femtosecond laser beam onto a 3-mm-thick sapphire plate. The time resolution in our fs experiments was ~150 fs. The TA signal is then analyzed by a silicon charge-coupled device (CCD; S11071-1104, Hamamatsu) with a monochromator (Acton 2358, Princeton Instrument) at 1 kHz enabled by a custom-built control board from Entwicklungsbuero Stresing. The signal-to-noise ratio in differential transmission was better than 5 × 10 −5 after accumulating and averaging 1000 pump-on and pump-off shots for each data point. The angle between the polarized pump and probe beams was set at the magic angle. For nanosecond TA spectroscopy, we used a sub-nanosecond laser (Picolo AOT MOPA, InnoLas) at 355 nm (pulse duration ~0.8 ns) to excite the samples. The laser was synchronized to the probe pulse with a desired delay by an electronic delay generator (SRS DG645, Stanford Research System). The diameters of the pump beam spots in fs and ns experiments were ~1 mm and 0.3 mm, respectively. The diameter of probe beam was ~0.2 mm. The pump fluence was kept ~100 μJ cm −2 in both experiments. The clusters dissolved in toluene were placed in 1 mm path length cuvettes for TA measurements. The optical density of samples at 550 nm was ~0.3.